Monoallelic expression ofTMPRSS2/ERGin prostate cancer stem cells While chromosomal translocations have a fundamental role in the development of several human leukaemias, their role in solid tumour development has been somewhat more controversial. Recently, it was shown that up to 80% of prostate tumours harbour at least one such gene fusion, and that the most common fusion event, between the prostate-specific TMPRSS2 gene and the ERG oncogene, is a critical, and probably early factor in prostate cancer development. Here we demonstrate the presence and expression of this significant chromosomal rearrangement in prostate cancer stem cells. Moreover, we show that in the prostate epithelial hierarchy from both normal and tumour tissues, TMPRSS2 transcription is subjected to tight monoallelic regulation, which is retained upon asymmetric division and relaxed during epithelial cell differentiation. The presence and expression of TMPRSS2/ERG in prostate stem cells would provide ERG-driven survival advantages, allowing maintenance of this mutated genotype. A dogma of cancer genetics stated until recently that chromosomal translocations did not have a role in epithelial solid tumours, but were of major significance in haematological malignancies [1] , [2] , for example the BCR-ABL translocation, which drives chronic myeloid leukaemia [3] . However, in 2005, Tomlins et al . [4] identified chromosomal translocations, which fused the promoter from the prostate-expressed, androgen responsive TMPRSS2 gene to two members of the ETS family: ERG and ETV1 . While multiple other gene fusions have now been demonstrated in prostate cancers (PCa) at lower frequencies [5] , the most commonly observed fusion remains that between TMPRSS2 and ERG (exon 1 to exon 4), which occurs in ~50% of all PCa. Unlike BCR-ABL , which results in a true fusion between two protein encoding sequences, the TMPRSS2/ERG fusion brings the potent oncogene ERG under the influence of the highly prostate and androgen-regulated TMPRSS2 gene promoter, resulting in the aberrant elevated expression of this ETS transcription factor. Clinically, the relevance of this common fusion to patient outcome remains unclear, as there is conflicting data about whether the presence of a fusion (or rearranged variations thereof) marks tumours with a good [6] or a bad [7] prognosis. According to the cancer stem cell (CSC) hypothesis, a rare population of tumour-initiating cells or CSCs exists, and has been demonstrated in both leukaemia and many solid tumours [8] . Furthermore, it has been proposed that it is this CSC population which is both responsible for the metastatic spread of cancers and comprises the therapy-resistant core of a tumour, driving tumour recurrences and relapse. Chromosomal translocations have been found frequently in leukaemic CSCs [2] , [9] , [10] , but only rarely in those of solid tumours. Although the presence of TMPRSS2/ERG has been detected in total PCa tissues, which are largely (>99%) composed of aberrantly differentiated, secretory luminal cell types, its presence, role and expression in the highly organized basal cell hierarchy of the prostate, and specifically CSCs, has not previously been studied. Were gene fusions like TMPRSS2/ERG , previously proposed to be tumour initiating, to be found and shown to be actively expressed in CSCs, it would provide further evidence for a hierarchical organization in this common solid tumour, and would establish the need to develop treatments to eliminate more than just the luminal populations targeted by the current treatments. Here we show that the TMPRSS2/ERG fusion is indeed present and expressed at both RNA and protein levels in the stem cell (SC) compartment from primary human PCas. Furthermore, the TMPRSS2 (and TMPRSS2/ERG fusion) expression is subject to a strong (but reversible) allelic exclusion and silencing during stem cell self-renewal and differentiation. Prostate CSCs contain the TMPRSS2/ERG gene fusion The basal compartment within the human prostate epithelial bilayer is composed of relatively undifferentiated cell types. This hierarchy of cell types can be segregated into a rare population of SC, responsible for the maintenance of the tissue itself, a rapidly proliferating and expanding transit-amplifying (TA) population and a population committed to differentiation, the committed basal (CB) cell type [11] , [12] . To study the TMPRSS2/ERG fusion within the basal hierarchy of cell types, we employed a primary culture method [13] , [14] to generate human prostate basal epithelial cultures, derived from human prostate tissue biopsies isolated directly from patient tumour samples. The presence of the TMPRSS2/ERG fusion at the genomic level in primary cultures and the positive control VCaP cell line ( Fig. 1a ) was established using two-colour break-apart fluorescence in-situ hybridization (FISH) [4] , [15] . This highlighted not only the fusion event in individual PCa patients, but also the heterogeneity of such primary cultures, where fusion-negative cells were also seen (left panel in Fig. 1a ). Although the proportion of TMPRSS2/ERG -positive/negative cells by FISH varied between individual cultures, transcription of fusion RNA, as detected by nested reverse transcription–PCR (RT–PCR) followed by Southern blot analysis ( Fig. 1b ) and confirmed by direct sequencing of the fusion breakpoint ( Fig.1c ), concurred with the FISH analysis. Each tumour had a unique fusion junction, as indicated by the variable molecular weight of the RT–PCR products in the top panels in Fig. 1b , and confirmed by direct sequencing. Unexpectedly, no clear correlation [16] was seen between TMPRSS2/ERG and TMPRSS2 expression. Additionally, in these primary cell cultures, wild-type TMPRSS2 expression levels did not always correspond to androgen receptor (AR) levels ( Fig. 1b ). 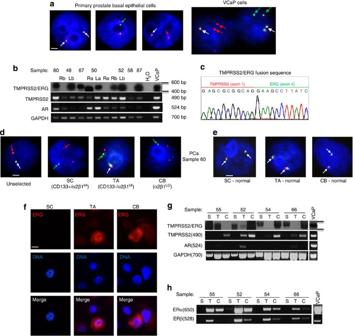Figure 1:TMPRSS2/ERGfusion in primary cultures and prostate CSCs. (a) Primary basal epithelial cultures derived from PCa tissues analysed by break-apart FISH for theTMPRSS2/ERGfusion. White arrows indicate normal, fusion-negative alleles. Green arrows indicate 5′-translocatedERGregions and red arrows highlight deletion events. The scale bars ina,bandecorrespond to 1 μm (b) Expression of theTMPRSS2/ERG(exon 1 to exon 4) fusion transcript detected with specific nested PCR primer sets for RT–PCR followed by Southern blotting with a fusion sequence-specific probe. Numbers above each image correspond to specific patients, lettering relates to needle biopsy locations (R, right; L, left; a, apex b, base). Expression of wild-typeTMPRSS2andARwere also investigated by RT–PCR to allow comparison with the fusion data.GAPDHexpression is a control for RNA integrity. PCR product sizes (in bp) are as indicated: forTMPRSS2/ERGthe molecular weight range is indicated (400–600 bp markers). (c) Confirmation of the unique fusion breakpoint by direct sequencing of RT–PCR products fromb. (d) FISH detection ofTMPRSS2/ERGfusion in total epithelial cell cultures fractionated into SC, TA and CB cell types using the CD133/α2β1 integrin selection process described previously13,14,15from patient 60 is shown. (e) Comparable FISH detection ofTMPRSS2andERGin a sample that does not contain a fusion (f) ERG protein detection (red stain) in selected cell populations from patient sample 60. A non-specific IgG primary antibody was used as a negative control and nuclei were counterstained with DAPI (blue). Scale bar, 5 μm. VCaP, Jurkat, BPH-1 and PC3 cell lines were used for truncated, wild-type or non-expressing ERG antibody controls (seeSupplementary Fig. S1). (g) Expression of theTMPRSS2/ERGfusion,TMPRSS2andARtranscripts in selected SC (S), TA (T) and CB (C) cell populations from four individual patient samples. Note variability of fusion transcript sizes. (h) Expression of oestrogen receptor isoform mRNA in comparable cell fractions fromg.GAPDHwas used as a control for RNA integrity and PCR product sizes (bp) are indicated in brackets next to gene names ingandh. Figure 1: TMPRSS2/ERG fusion in primary cultures and prostate CSCs. ( a ) Primary basal epithelial cultures derived from PCa tissues analysed by break-apart FISH for the TMPRSS2/ERG fusion. White arrows indicate normal, fusion-negative alleles. Green arrows indicate 5′-translocated ERG regions and red arrows highlight deletion events. The scale bars in a , b and e correspond to 1 μm ( b ) Expression of the TMPRSS2/ERG (exon 1 to exon 4) fusion transcript detected with specific nested PCR primer sets for RT–PCR followed by Southern blotting with a fusion sequence-specific probe. Numbers above each image correspond to specific patients, lettering relates to needle biopsy locations (R, right; L, left; a, apex b, base). Expression of wild-type TMPRSS2 and AR were also investigated by RT–PCR to allow comparison with the fusion data. GAPDH expression is a control for RNA integrity. PCR product sizes (in bp) are as indicated: for TMPRSS2/ERG the molecular weight range is indicated (400–600 bp markers). ( c ) Confirmation of the unique fusion breakpoint by direct sequencing of RT–PCR products from b . ( d ) FISH detection of TMPRSS2/ERG fusion in total epithelial cell cultures fractionated into SC, TA and CB cell types using the CD133/α2β1 integrin selection process described previously [13] , [14] , [15] from patient 60 is shown. ( e ) Comparable FISH detection of TMPRSS2 and ERG in a sample that does not contain a fusion ( f ) ERG protein detection (red stain) in selected cell populations from patient sample 60. A non-specific IgG primary antibody was used as a negative control and nuclei were counterstained with DAPI (blue). Scale bar, 5 μm. VCaP, Jurkat, BPH-1 and PC3 cell lines were used for truncated, wild-type or non-expressing ERG antibody controls (see Supplementary Fig. S1 ). ( g ) Expression of the TMPRSS2/ERG fusion, TMPRSS2 and AR transcripts in selected SC (S), TA (T) and CB (C) cell populations from four individual patient samples. Note variability of fusion transcript sizes. ( h ) Expression of oestrogen receptor isoform mRNA in comparable cell fractions from g . GAPDH was used as a control for RNA integrity and PCR product sizes (bp) are indicated in brackets next to gene names in g and h . Full size image As culture heterogeneity could explain this, we next analysed individual cell populations within the basal primary epithelial cultures, derived from CSCs, by fractionating these mixed epithelial populations using a combination of CD133 expression and rapid adhesion to type 1 collagen (high α2β1 integrin expression) [14] , [17] , [18] . FISH analysis of fractionated cell cultures isolated from known TMPRSS2/ERG -positive samples confirmed the presence of the fusion in all fractionated populations, an example of which (sample 60) is shown in Fig. 1d , although again some fusion-negative epithelial cells were always present ( Fig. 1e ). Immunofluorescence analysis of subsequent ERG protein expression in corresponding fractionated cell populations from the above sample gave intriguing results ( Fig. 1f ). Although sample 60 had presented with fusion-positive cells, by FISH, in all populations, ERG protein expression was limited to the TA and CB cell types. Reassuringly, ERG expression was not observed in all cells within the TA and CB populations, correlating with the presence of fusion-negative cells observed within the FISH experiments. Analysis of control cell lines, Jurkat, VCaP (± 10 nM R1881), BPH-1 and PC3 ( Supplementary Fig. S1a ), which also showed the expected potent upregulation of ERG expression in VCaP cells after androgen treatment further validated these data. In addition, TMPRSS2/ERG -negative, primary prostate basal epithelial cultures (sample 25, from BPH and sample 58, a Gleason 7 cancer) had no detectable ERG protein in their selected cell populations ( Supplementary Fig. S1b,c ). RT–PCR analysis of both TMPRSS2/ERG and wild-type TMPRSS2 transcription in fractionated cell populations from a number of known fusion-positive primary cultures, gave results similar to those previously reported [19] , whereas expression of TMPRSS2/ERG was detectable in all basal cell subtypes from the various cultures, including prostate CSCs ( Fig. 1g ). However, as with ERG protein expression, the TMPRSS2/ERG transcript was not always detectable in all of the selected cell populations isolated from a single sample, even after Southern blot enhancement of the signals (top lane Fig. 1g ). This implied extremely tight regulation of transcription. The patterns of expression varied greatly between samples; for example, TMPRSS2/ERG expression was detected in all populations isolated from sample 52 but was absent in the CB population of 55 (both from Gleason 8 (4+4) tumour tissues). In contrast, samples 54 and 66 had matching fusion transcript patterns where the CSC population expressed the fusion, but the TA cell population had completely switched off expression, which was restored in the CB cell population ( Fig. 1g ). These cultures were derived from Gleason 9 (5+4) and Gleason 7 (3+4) tumours, respectively ( Table 1 ). Indeed, this pattern of fusion expression implicated additional mechanisms for the regulation of TMPRSS2/ERG within the prostate basal cell hierarchy, where its expression could be sequentially switched from active to silent or vice versa during differentiation. In several samples, the data implied an allelic switch between the TMPRSS2 promoter in the fused allele and the unfused allele during differentiation. Our data also suggested that regulation of TMPRSS2 , and more compellingly TMPRSS2/ERG , in the prostate basal epithelium was not solely due to the actions of AR ( Fig. 1b ), or indeed oestrogen receptors (ERα and β) in the CSC fraction ( Fig. 1h ; ref. 20 ). Androgen receptor expression was either absent in the SC fraction, but increased (with TMPRSS2 expression) as the cells committed to differentiation in CB cells, while ER transcription was confined to the TA and CB populations, highest in the TA populations and showing a broadly reciprocal pattern of expression to that of the AR . Table 1 TMPRSS2/ERG fusion status of patient biopsies. Full size table To give a more complete impression of TMPRSS2/ERG presence and expression within the prostate basal epithelial cell hierarchy, complete data ( Fig. 2 ) of expression from an individual PCa (Gleason 6) sample (50 La) are shown. Immunohistochemical analysis of paraffin-embedded tissue sections showed ERG overexpression (arrowed in Fig. 2a ). The presence of the TMPRSS2/ERG fusion was confirmed in the resulting primary epithelial culture and the hierarchical cell populations isolated from it by FISH ( Fig. 2b ). The fusion transcript was also detectable by RT–PCR and Southern blot within the total population ( Figs 1b and 2e ). ERG protein analysis within the selected cell populations showed fusion expression in the SC and CB cell populations, as well as its extremely low levels or complete absence in the TA cells ( Fig. 2c ), similar to the RNA transcript expression patterns of samples 54 and 66 ( Fig. 1g ). When clonal cell populations, derived from single CSCs isolated from the fusion-positive sample 50 La, were analysed by FISH ( Fig. 2d ), the TMPRSS2/ERG fusion was found to be present in 3/5 clones investigated. Subsequent nested RT–PCR/Southern blot analysis correlated with the FISH data, highlighting the transcription of fusion RNA only in the FISH-positive clones. This confirmed that CSCs containing and expressing the TMPRSS2/ERG fusion were capable of founding new colony growth from single cells (clonogenicity: a fundamental SC property) and that fusion gene presence and expression was clonally maintained during colony development and subsequent epithelial cell differentiation. 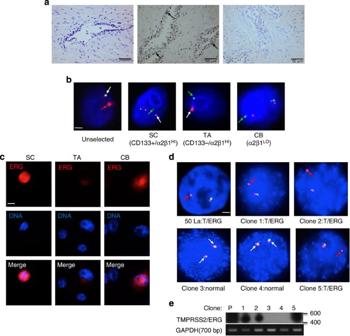Figure 2:TMPRSS2/ERGexpression in tumour tissues and cell cultures. (a) Immunohistochemical analysis of paraffin-embedded tissue sections from patient 50 La (counterstained with haematoxylin): No antibody (left panel) and ERG-positive (centre panel) and negative immunohistochemistry control (right panel) are shown.TMPRSS2/ERG-positive cells are indicated using black arrows. (b) FISH images indicating the presence of theTMPRSS2/ERGfusion in unselected and selected (SC, TA and CB) cell populations from patient sample 50 La. White arrows indicate normal, fusion-negative alleles. Green arrows indicate 5′-translocated ERG regions and red arrows highlight deletion events. Scale bar, 1 μm. (c) ERG protein analysis in selected cell populations from patient 50 La. VCaP, Jurkat, BPH-1 and PC3 cell lines were used for truncated, wild-type or non-expressing ERG antibody controls (seeSupplementary Fig. S1). Scale bar, 5 μm. (d) Colonies derived from single prostate cancer stem cells isolated directly from the 50 La parental culture analysed for the maintenance of theTMPRSS2/ERGfusion event throughout differentiation by FISH. FISH images from single nuclei representative of five individual clones and their respective parental culture (SC only) are shown. Scale bar represents 1 μm. (e) RT–PCR/Southern blot image ofTMPRSS2/ERGfusion expression from parent culture (50 La) and individual clones. Note the lack of fusion expression in fusion-negative colonies ind.GAPDHwas used as a control for RNA integrity and PCR product sizes (in bp) are as indicated. Figure 2: TMPRSS2/ERG expression in tumour tissues and cell cultures. ( a ) Immunohistochemical analysis of paraffin-embedded tissue sections from patient 50 La (counterstained with haematoxylin): No antibody (left panel) and ERG-positive (centre panel) and negative immunohistochemistry control (right panel) are shown. TMPRSS2/ERG -positive cells are indicated using black arrows. ( b ) FISH images indicating the presence of the TMPRSS2/ERG fusion in unselected and selected (SC, TA and CB) cell populations from patient sample 50 La. White arrows indicate normal, fusion-negative alleles. Green arrows indicate 5′-translocated ERG regions and red arrows highlight deletion events. Scale bar, 1 μm. ( c ) ERG protein analysis in selected cell populations from patient 50 La. VCaP, Jurkat, BPH-1 and PC3 cell lines were used for truncated, wild-type or non-expressing ERG antibody controls (see Supplementary Fig. S1 ). Scale bar, 5 μm. ( d ) Colonies derived from single prostate cancer stem cells isolated directly from the 50 La parental culture analysed for the maintenance of the TMPRSS2/ERG fusion event throughout differentiation by FISH. FISH images from single nuclei representative of five individual clones and their respective parental culture (SC only) are shown. Scale bar represents 1 μm. ( e ) RT–PCR/Southern blot image of TMPRSS2/ERG fusion expression from parent culture (50 La) and individual clones. Note the lack of fusion expression in fusion-negative colonies in d . GAPDH was used as a control for RNA integrity and PCR product sizes (in bp) are as indicated. Full size image Monoallelic expression of TMPRSS2/ERG in prostate CSCs Within the fractionated epithelial cells, we frequently observed an imbalance between the expression of the fusion allele and its unfused homologue ( Fig. 1g ), which was not apparent in total cell populations ( Fig. 1b ). As all fractions contained fusion-positive cells, this implied an allelic exclusion or imprint, as seen for other genes in embryonal tumours, the developing embryo and more recently in adult lung tissue SCs [21] . We now wished to test whether allelic restriction was driven by the fusion event, or was a property of TMPRSS2 in the hierarchical epithelial populations. To achieve this, we determined the frequency of single-nucleotide (G/A) polymorphisms (SNP) in exon 6 of TMPRSS2 by pyrosequencing ( Fig. 3a ) to identify the expressed alleles (strategy shown in Fig. 3b ). From another twenty, predominantly fusion-negative primary basal cell cultures ( Table 2 ), which expressed TMPRSS2 as detected by RT–PCR ( Fig. 3c ), five (25%) were genotypically heterozygous for the commonest SNP (position 264). The sensitivity of the strategy is shown in Fig. 3d where A and G homozygotes were mixed in varying proportions. The results on analysis of total epithelial cell populations in the five heterozygotes ( Fig. 3e ) revealed some preferential allelic expression, with sample 8 expressing almost only the G allele ( Fig. 3e ). 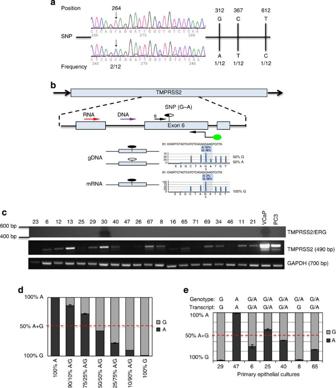Figure 3: Allelic expression ofTMPRSS2in primary epithelial cultures. (a) Identification of SNP (rs12329760) in exon 6 (bp264) ofTMPRSS2is shown, together with other less frequent SNPs. (b) Diagrammatic overview of the pyrosequencing analysis of SNP (rs12329760) in exon 6 ofTMPRSS2. Biotinylated primer sets were used to amplify DNA and RNA independently. The purified PCR amplification products were independently subjected to pyrosequencing using the indicated sequencing primers. gDNA, genomic DNA. (c) Screening of total epithelial cell cultures from the patients indicated by numbers at the top of the figure to identifyTMPRSS2–expressing heterozygotes for analysis. The VCaP and PC3 cell lines were used as positive and negative controls, respectively, for RT–PCR. PCR product size is indicated at the left of the figure (in bp). (d) Evaluation of the sensitivity of the allele-specificity assay by mixing of G and A homozygotes in the proportions indicated. Indande, the genotype and RNA transcript are indicated above the graph with a single G or A representing a homozygous sample and a G/A denoting a heterozygous sample. Error bars signify s.d. of three independent experimental replicas. The results confirmed a confidence interval of ±5% for allele quantification. (e) Allelic expression analysis of total RNA from cultured unfractionated epithelial cells of two homozygotes and five heterozygotes, indicating a modest allelic imbalance in expression ofTMPRSS2. Figure 3: Allelic expression of TMPRSS2 in primary epithelial cultures. ( a ) Identification of SNP (rs12329760) in exon 6 (bp264) of TMPRSS2 is shown, together with other less frequent SNPs. ( b ) Diagrammatic overview of the pyrosequencing analysis of SNP (rs12329760) in exon 6 of TMPRSS2 . Biotinylated primer sets were used to amplify DNA and RNA independently. The purified PCR amplification products were independently subjected to pyrosequencing using the indicated sequencing primers. gDNA, genomic DNA. ( c ) Screening of total epithelial cell cultures from the patients indicated by numbers at the top of the figure to identify TMPRSS2 –expressing heterozygotes for analysis. The VCaP and PC3 cell lines were used as positive and negative controls, respectively, for RT–PCR. PCR product size is indicated at the left of the figure (in bp). ( d ) Evaluation of the sensitivity of the allele-specificity assay by mixing of G and A homozygotes in the proportions indicated. In d and e , the genotype and RNA transcript are indicated above the graph with a single G or A representing a homozygous sample and a G/A denoting a heterozygous sample. Error bars signify s.d. of three independent experimental replicas. The results confirmed a confidence interval of ±5% for allele quantification. ( e ) Allelic expression analysis of total RNA from cultured unfractionated epithelial cells of two homozygotes and five heterozygotes, indicating a modest allelic imbalance in expression of TMPRSS2 . Full size image Table 2 Single-nucleotide polymorphisms in TMPRSS2 gene from individual patients. Full size table Following fractionation, while the DNA SNP profile of the SC, TA and CB cells matched their respective total cell cultures, the transcript data now showed a substantial preferential allelic expression of either G or A polymorphisms, particularly in the SC population, from 4/5 heterozygotes ( Fig. 4a ). Promoter methylation studies within selected basal cell populations from fusion-positive and -negative samples ( Fig. 4b ) could not explain this allelic imbalance. In addition, preferential TMPRSS2 expression did not correlate with a specific SNP, indicating that the observed monoallelic expression was defined at the transcriptional level and was not due to allelic mRNA instability. 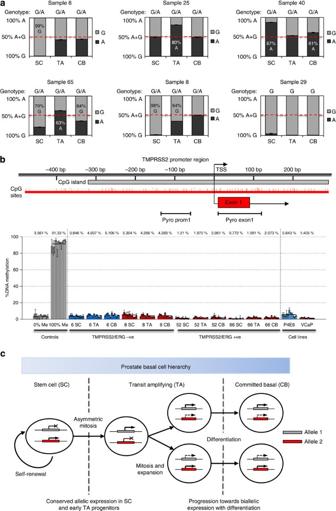Figure 4: Preferential allelic expression ofTMPRSS2. (a) Graphs show the RNA data obtained from CD133/α2β1 integrin selected sub-populations (SC, TA and CB cells) for the five heterozygotes (6, 25, 40, 65 and 8) and a single homozygous control sample (29). The lettering above the graph indicates the genotype for each sub-population as previously stated. Percentages within individual columns highlight the allelic preference (%) in RNA transcripts directly quantified from the pyrosequencing trace. The dashed red line at 50% indicates samples with no allelic preference of expression. Error bars signify the s.d. of three independent experimental replicas. (b) Analysis of expression-related genome methylation in the promoter region of theTMPRSS2gene fromTMPRSS2-expressing and non-expressing epithelial cells fractionated from primary epithelial cultures. Top panel illustrates the distribution of CpG islands in the promoter proximal regions and the position of the segments used in the pyrosequencing analysis. Lower panel shows the % methylation of the Pyroprom1 fragment (there were no significant changes with the Pyroexon1 fragment—not shown). Positive and negative controls run in parallel are shown at the left of the figure. No significant increase in promoter methylation, which could account for lack ofTMPRSS2expression was detected. (c) Schematic representation ofTMPRSS2preferential allelic expression patterns identified in the human prostate basal cell hierarchy12. Monoallelic expression from theTMPRSS2promoter is present in the stem and early transit-amplifying cell types. As these cell types commit to differentiation, transcription of the ‘silent’ allele is initiated resulting in bi-allelic gene expression in the CB cell types. Figure 4: Preferential allelic expression of TMPRSS2 . ( a ) Graphs show the RNA data obtained from CD133/α2β1 integrin selected sub-populations (SC, TA and CB cells) for the five heterozygotes (6, 25, 40, 65 and 8) and a single homozygous control sample (29). The lettering above the graph indicates the genotype for each sub-population as previously stated. Percentages within individual columns highlight the allelic preference (%) in RNA transcripts directly quantified from the pyrosequencing trace. The dashed red line at 50% indicates samples with no allelic preference of expression. Error bars signify the s.d. of three independent experimental replicas. ( b ) Analysis of expression-related genome methylation in the promoter region of the TMPRSS2 gene from TMPRSS2 -expressing and non-expressing epithelial cells fractionated from primary epithelial cultures. Top panel illustrates the distribution of CpG islands in the promoter proximal regions and the position of the segments used in the pyrosequencing analysis. Lower panel shows the % methylation of the Pyroprom1 fragment (there were no significant changes with the Pyroexon1 fragment—not shown). Positive and negative controls run in parallel are shown at the left of the figure. No significant increase in promoter methylation, which could account for lack of TMPRSS2 expression was detected. ( c ) Schematic representation of TMPRSS2 preferential allelic expression patterns identified in the human prostate basal cell hierarchy [12] . Monoallelic expression from the TMPRSS2 promoter is present in the stem and early transit-amplifying cell types. As these cell types commit to differentiation, transcription of the ‘silent’ allele is initiated resulting in bi-allelic gene expression in the CB cell types. Full size image The products of tumour-initiating fusion genes in haematopoietic CSC such as TEL-AML1 (or ETV6/RUNX1 ) in childhood leukaemia can influence both self-renewal and survival in undifferentiated cell populations [2] , [22] . Indeed, it has been proposed that the fusion gene is responsible for repression of multiple gene sets, maintaining the leukaemic initiating pool, in the absence of any requirement for subsequent mutagenic changes in cells within tumour bulk [22] . Based on the data we have presented, we can now propose a similar role for TMPRSS2/ ERG in the early stages of human PCa. As shown in haematopoietic CSCs [23] , [24] and more recently in a prostate transgenic mouse model [25] , ERG expression can indeed influence self-renewal and maintenance of the stem cell pool. As the SC are likely to have a longer life span (together with their immediate progeny the TA cells) they have been proposed as the cells most likely to accumulate the necessary genetic (and epigenetic) changes required to escape niche dependence and normal growth/survival controls. The aberrant expression of ERG would, therefore, provide a means of short-term expansion of a primarily quiescent population, necessary to establish any mutations. Thus, the presence and expression of TMPRSS2/ERG , which we have observed in prostate CSCs from ‘successful’ cancers would provide selective ERG -driven advantages over fusion-negative counterparts in the SC compartment. Increased, deregulated expression of ERG in SC could also have considerably different consequences to that proposed in fully differentiated proliferating luminal cells from PCas. The experimental approach of tumour fractionation that we have employed has resulted in the identification of potential new targets for tumour therapy [26] , [27] . In an extract of total primary tumour tissues, the scarcity of the CSC population and the mRNA from highly expressed genes for secretory proteins such as prostate-specific antigen and prostatic acid phosphatase and luminal structural proteins such as cytokeratins which predominate in expression signatures [26] means that the CSC expression signature is masked. Therefore, specific gene expression from the small percentage of CSCs would not be apparent, but it is the rare CSCs which are responsible for tumour induction in immunocompromised mice [19] . However, the primary culture approach can be criticized as it produces only cells capable of expansion in vitro , where the selective pressures imposed by growth matrix (collagen) and medium (serum-free stem cell factor enriched medium) certainly differ from those in the original tissue. Despite surgical precision in our biopsy of the original tumours, the ultimate cell population remains heterogeneous, and contains variable proportions of non-malignant cells. This heterogeneity was apparent upon isolation and characterization of individual cell clones, each originating from an original single clonogenic stem cell for example, in Fig. 2d only 3/5 of such colonies studied in detail (from biopsy 50) contained and expressed the TMPRSS2/ERG fusion. After prolonged culture of such primary epithelium, we had previously observed changes in biological behaviour, and in these experiments it became apparent that the TMPRSS2/ERG -containing populations were at a selective disadvantage, and were eliminated from the populations after repeated passage in long-term culture. This is in agreement with the relative scarcity of TMPRSS2/ERG fusions in established cell lines, despite its reported presence in 50% of prostate tumours [4] . Our data also pose further questions about the factors, which influence TMPRSS2/ERG expression when it is detectable in the SC compartment. As we have shown here and in previous publications [17] that, as AR and ER expression at the mRNA level (and also at protein level [19] ) is barely detectable/undetectable, TMPRSS2/ERG expression is unlikely to be controlled by sex hormones in SC. Hormonal control was clearly evident ( Fig. 1 ) when the epithelial cells commit to differentiation (in the CB cells), but because a gene can be regulated by sex hormones does not mean that it can only be so regulated. As shown in Fig. 4b , TMPRSS2 expression in tissues and SC is also unlikely to be silenced by a global or indeed regional genome methylation, as implied by some previous studies in established cell lines, following a pattern we have recently reported for the tight control of transcription of the CD133 gene [28] . In contrast to our observed expression of TMPRSS2/ERG in the stem cell compartment of tumours, were the fusion to occur on the silenced allele in a precancerous state, this would have no phenotypic consequences, but could affect more differentiated progeny if and when the allelic suppression is relaxed ( Fig. 4c ), In cells of a more differentiated phenotype, the pleiotrophic effects of ectopic ERG expression would include the induction of both cell proliferation and the generation of further aneuploidy [29] . Allelic silencing of mutationally activated cell fate-altering loci in SCs would allow long-term accumulation of mutations, maintaining the mutated genotype even when their oncogene-expressing daughter cells were deleted by local microenvironmental influences such as immune responses, and cell protective or repair mechanisms. This is also reminiscent of the situation with TEL-AML1 expression leukaemic stem cells. However, if the local cellular microenvironment selected in favour of a particular gene set, for example, as a resistance response to hormone therapies in PCa [27] , then reversal of allelic silencing would provide a mechanism whereby both therapy resistance and even ‘pre-tumour’ progression [30] could rapidly occur. The importance of the ERG -activating rearrangement in the development of PCa has been demonstrated by tracking of the fused allele from positive high-grade prostatic intraepithelial neoplasia to development of primary tumours [31] , [32] . Additional studies have also matched TMPRSS2/ERG fusions in castration-resistant PCa lymph node metastases to localized primary tumours [33] , [34] , implying that early clonal expansion from a more primitive stem cell is indeed prevalent in PCa. Any lack of correlation between the presence of TMPRSS2/ERG and the unfavourable outcome of PCa [6] would suggest that, although ERG protein has a potent cancer-inductive power, the selection processes during and after hormone response therapy, which result in fatal castration-resistant PCa, would require other genetic and epigenetic changes. It seems that the best chance of exploiting TMPRSS2/ERG as a therapeutic target probably is, therefore, at the precastration stage of PCa treatment. As such, we now need to understand the underlying regulatory mechanisms involved in the expression of TMPRSS2/ERG , and its functional activity, in the SC and basal cell populations. We also need to assess the extent of allelic silencing as a mechanism for the control of the expression of other fate-altering genes in primary human cancers, rather than in cell lines where phenotypes and proportions of different epithelial cell types are more variable. Tissue collection, isolation and culture of prostate epithelial cells Human prostate tissue was obtained from patients undergoing radical prostatectomy, by directed needle biopsy, and transurethral resection of the prostate for either PCa or BPH. PCa or BPH diagnosis was confirmed by histological examination of representative adjacent fragments. Tissues were disaggregated and cultured as described previously [13] , [14] . Basal epithelial cultures were further fractionated on the basis of rapid adhesion to type 1 collagen and their expression of the CD133 surface marker using magnetic activated cell sorting (MACS) microbeads linked to anti-human CD133, according to the manufacturer’s instructions (Miltenyi Biotec) [17] . Cell lines: VCaP (kindly provided by Dr K. Pienta, University of Michigan) were maintained in R10 medium (RPMI1640 (Gibco)+10 mM HEPES+2 mM glutamine+10% fetal calf serum). PC3 cells were grown in H7 medium (Ham’s F12 (Gibco)+2 mM glutamine+7% fetal calf serum). Reverse transcription–PCR RNA was extracted using the RNeasy mini kit (Qiagen) following the manufacturer's instructions. The RNA was reverse transcribed using random hexamers (Invitrogen) and reverse transcriptase (Superscript III, Invitrogen). The TMPRSS2/ERG fusion transcript was detected by nested PCR with specific primers; first step, forward 5′-CGCGAGCTAAGCAGGAGGC-3′ and reverse 5′-GGCGTTGTAGCTGGGGGTGAG-3′; second step, forward 5′-GGAGCGCCGCCT GGAG-3′ and reverse 5′-CCATATTCTTTCACCGCCCACTCC-3′; (Invitrogen). Variably sized nested PCR products between 450 and 600 bp were produced in different human PCa samples (depending on the translocation breakpoint). Nested PCR conditions were: first step; 94 °C for 30 s followed by 35 cycles of 94 °C for 20 s and 68 °C for 1 min followed by 68 °C for 7 min, second step; 94 °C for 30 s, 35 cycles of 94 °C for 20 s, 66 °C for 10 s and 68 °C for 1 min followed by 68 °C for 7 min. PCR analysis of TMPRSS2 , AR , ERα , ERβ and GAPDH (glyceraldehyde 3-phosphate dehydrogenase) was carried out in a final volume of 25 μl using Platinum Taq DNA polymerase (Invitrogen). Primers to detect the presence of these genes were as follows: TMPRSS2 ; forward 5′-TTTGAACTCAGGGTCACCAC-3′, reverse 5′-CCTCTGAGATGAGTACATCTG-3′, annealing temperature 54 °C; AR ; forward 5′-CGAAATGGGCCCCTGGATGGATAG-3′, reverse 5′-AGTCGGGCTGGTTGTTGTCGTGTC-3′, annealing temperature 58 °C; ERα ; forward 5′-TACTGCATCAGATCCAAGGG-3′, reverse 5′-ATCAATGGTGCACTGGTTGG-3′, annealing temperature 55 °C; ERβ ; forward 5′-TGAAAAGGAAGGTTAGTGGGAACC-3′, reverse 5′-TGGTCAGGGACATCATCATGG-3′, annealing temperature 58 °C; GAPDH ; forward 5′-AAGGTGAAGGTCGGAGTCAA-3′, reverse 5′-GGACACGGAAGGCCATGCCA-3′, annealing temperature 58 °C. PCR conditions were 94 °C for 2 min followed by 30 cycles (25 for GAPDH) of 94 °C for 30 s, appropriate annealing temperature for 30 s and 72 °C for 30 s followed by a final extension of 72 °C for 5 min. PCR products were separated by electrophoresis through a 1.0% (w/v) agarose GelRed (Invitrogen) stained gel for 1 h at 80 V. PCR products were visualized using a Gene Genius bio-imaging system. Southern blotting of RT–PCR products A PCR product, derived from the VCaP cell line, corresponding to TMPRSS2 exon 1 fused to exon 4 of ERG was cloned and labelled with digoxigenin (DIG) using the PCR DIG Probe Synthesis kit (Roche) following the manufacturer’s protocol. Nested RT–PCR products were run on a 1.0% (w/v) agarose gel and transferred to a positively charged nylon membrane (Roche) overnight. Hybridization was carried out using DIG Easy Hyb buffer (Roche) containing the labelled probe at 50 °C followed by blocking (1:100 dilution Roche blocking solution). Bands were detected by incubating blots with anti-DIG alkaline phosphatase conjugated antibody (Roche) followed by addition of CSPD (Roche). Bands were visualized by exposure to X-ray film. Fluorescence in-situ hybridization Break-apart FISH was carried out as previously described [4] , [15] . Cells were fixed in 3:1 methanol: acetic acid and attached to 3-aminopropyltriethoxysilane-coated slides (Superfrost Plus, VWR). Slides were aged for at least 1 week at −20 °C. Before hybridization with labelled probes (Empire Genomics), slides were equilibrated in 2 × SSC buffer followed by denaturation in a 70% formamide solution for 5 min at 73 °C. Slides were then dehydrated in an ethanol series (70–85–100%—precooled to −20 °C) and allowed to air dry. The probe mix (9 μl hybridization buffer+1μl probe) was added to the slide, covered with a coverslip and sealed with Cowgum. Slides were placed in a hybridization chamber and denatured for 5 min at 73 °C followed by incubation at 37 °C for 16 h. The coverslip was then removed and slides were washed and mounted in Vectashield+4',6-diamidino-2-phenylindole (DAPI) (Vector Laboratories) and fresh coverslip added. Slides were examined on a Nikon Eclipse TE300 microscope. Images were captured using Volocity software. Pyrosequencing RNA was extracted and reverse transcribed as above. DNA was extracted using the DNA blood and tissue kit (Qiagen) and the QIamp DNA micro kit (Qiagen) for SC samples. Allelic analysis The TMPRSS2 exon 6 SNP region was amplified from both DNA and RNA ( Fig. 3 ) using specific primer sets: DNA forward; 5′-AGGTGACAGAGCGAGACTCC-3′, RNA forward; 5′-AACTGGTGTGATGGCGTGTC-3′, biotinylated reverse; 5′-GCCCGTAGTTCTC GTTCCA-3′. PCR conditions were 95 °C for 5 min followed by 45 cycles of 94 °C for 30s, 58 °C for 30s and 72 °C for 20s followed by a final extension of 72 °C for 10 min. Products were analysed with the PyroMark Q24 system (Qiagen) using a specific sequencing primer; 5′-GGACCAAACTTCATCCTT-3′. Data were evaluated with PyroMark Q24 software. Methylation analysis The TMPRSS2 promoter sequences were amplified by PCR by specific primers for two regions within the CpG island, Pyroprom1 (forward; 5′-GTTGAGTTAGGTAGGGAATT-3′ and reverse; 5′-CCCCTAACTCTCCCTTTAATCTCAAAA-3′): PCR product 157 bp or Pyroexon1 (forward; 5′-GGGTG TAGTTTTGGATTTTGGGATAT-3′ and reverse; 5′-AAACCCCCAAATTCCCCTCCC-3′): PCR product 210 bp and sequenced using the PyroMark Q24 system (Qiagen) using specific sequencing primers (Pyroprom1; 5′-CCAAAACCACACCCCC-3′ and Pyroexon1; 5′-AGATTAAAGAGAGAGTT AGG-3′). Data were analysed using PyroMark Q24 software. Immunohistochemistry Formalin-fixed paraffin-embedded prostate tissue sections (5 μm) were processed with the following procedure. Slides were baked (20 min at 45 °C) then dewaxed in Xylene. Hydration through an ethanol series to tap water was followed by antigen retrieval in a sodium citrate buffer. Slides were blocked in 20% normal goat serum for 15 min. Slides were incubated for 1 h with rabbit monoclonal anti-ERG (clone EPR3864, 1:100 dilution; Abgent Inc.), washed and incubated with a goat anti-rabbit biotin-conjugated antibody for 30 min (1:200 dilution; Dako). Slides were further incubated with a streptavidin-HRP-conjugated antibody (1:100 dilution; Thermo scientific) for 30 min before detection with a DAB (3, 3'-diaminobenzidine, Sigma) for 7 min. Slides were weakly counterstained with haematoxylin and dehydrated by ethanol series before coverslips were mounted in DPX (Fluka). Images were obtained using an Olympus UC30 microscope with Cell B software. Immunofluorescence VCaP (±10 nM R1881 for 24 h), BPH-1, PC3, Jurkat and primary prostate epithelial cells, selected where appropriate into SC, TA and CB cell populations, were seeded onto 8-well chamber slides (BD Biocoat) and allowed to adhere for 24 h. All slides were washed in PBS before fixation in 4% paraformaldehyde for 15 min before two further PBS washes. Initial permeabilisation was with 0.2% Triton X-100 for 20 min followed by 3 × 5 min washes in PBS. Slides were then further treated with 0.5% NP40 for 20 min, followed by 3 × 5 min washes in PBS. Slides were blocked with 2% BSA+1% goat serum for 1 h before the addition of primary antibody (anti-ERG, clone ab96697, Abcam) diluted 1:100 in 3% BSA/PBS overnight at 4 °C. Slides were washed 3 × 5 min with 0.5% BSA+0.175% tween 20, before incubation in secondary antibody (alexa-fluor 488, diluted 1:1000 in 3% BSA/PBS, Molecular probes) for 45 min. Slides were again washed 3 × 5 min with 0.5% BSA+0.175% tween 20 and once in PBS only, before mounting coverslips with Vectashield+DAPI mountant (Vector laboratories). Slides were examined on a Nikon Eclipse TE300 microscope. Images were captured using Volocity software. How to cite this article: Polson, E. S. et al . Monoallelic expression of TMPRSS2/ERG in prostate cancer stem cells. Nat. Commun. 4:1623 doi: 10.1038/ncomms2627 (2013).